Genetic pathways for differentiation of the peripheral nervous system in ascidians Ascidians belong to tunicates, the sister group of vertebrates. Peripheral nervous systems (PNSs) including epidermal sensory neurons (ESNs) in the trunk and dorsal tail regions of ascidian larvae are derived from cells adjacent to the neural plate, as in vertebrates. On the other hand, peripheral ESNs in the ventral tail region are derived from the ventral ectoderm under the control of BMP signalling, reminiscent of sensory neurons of amphioxus and protostomes. In this study, we show that two distinct mechanisms activate a common gene circuit consisting of Msx , Ascl.b , Tox , Delta.b and Pou4 in the dorsal and ventral regions to differentiate ESNs. Our results suggest that ventral ESNs of the ascidian larva are not directly homologous to vertebrate PNSs. The dorsal ESNs might have arisen via co-option of the original PNS gene circuit to the neural plate border in an ancestral chordate. Peripheral nervous systems (PNSs) include sensory neurons. In vertebrate embryos, PNSs arise from the border of the neural plate [1] , [2] , [3] , [4] . Cranial neural crest cells and placodes contribute to the cranial PNS, whereas the caudal PNS is thought to be derived only from neural crest cells. In anamniote embryos, additional mechanosensory neurons called Rohon-Beard sensory neurons are also formed from the neural plate border [5] , [6] . On the other hand, in cephalochordates, the most basal chordate group, in which no neural crest cells or placodes have been identified, epidermal sensory neurons (ESNs) are found along the entire length of larval and adult bodies [7] , [8] . These ESNs are derived from the ventral ectodermal region of neurula embryos. Ciona intestinalis is a member of the tunicates, the closest relatives of vertebrates. In this species, the palps, which contain sensory neurons and differentiate at the anterior end of the larva, are derived from the anterior border of the neural plate [9] . By contrast, the pigment cells, which differentiate in the brain, are derived from the anterolateral border of the neural plate [10] . Indeed, the anterior and anterolateral borders of the neural plate are suggested to be a rudimentary placode and primitive neural crest, respectively [11] , [12] , [13] , [14] , [15] . The posterolateral border of the neural plate gives rise to the dorsal row of the tail nerve cord and dorsal epidermis, and ESNs are differentiated from this dorsal epidermis ( Supplementary Fig. 1 ) [16] . In addition to these PNS neurons, the ascidian larva has ESNs in the ventral region of the tail. A cell lineage analysis revealed that this ventral region is not derived from the border of the neural plate [16] . The posterolateral border of the neural plate is induced at the 32-cell stage in a process coordinated by four signalling molecules [17] , [18] , [19] , [20] , [21] , [22] . Fgf9/16/20 signalling activates Otx and Nodal in a cell pair called b6.5 ( Supplementary Fig. 1 ). Signalling of EfnA.d (formerly EphrinA-d, renamed according to a recently published nomenclature rule [23] ), Gdf1/3-r (called Gdf1/3-like or Orphan TGFβ 2) and Admp (a bone morphogenetic protein (BMP)-related ligand) negatively regulates expression of Otx and Nodal . The Otx transcription factor and Nodal signalling cooperatively activate expression of Msx (formerly Msxb ) and Delta.b (formerly Delta-like or Delta2 ) [24] , [25] . On the other hand, the ventral ESNs are induced by Admp, which is expressed in the endoderm lining the ventral ectodermal region [16] , [25] . Although the detailed molecular mechanisms remain to be elucidated, the ventral ESN lineage cells also express Msx and Delta.b [16] , [26] . In neural induction of vertebrate embryos, BMPs negatively regulate neural fate, FGFs positively induce neural fate [27] , [28] , [29] , [30] , [31] and neural crest and placodes arise from a region at the border of the neural plate [32] . On the other hand, in cephalochordate embryos, BMPs positively induce ESNs [33] . BMP signalling also positively regulates PNS formation in protostomes, including flies and annelids [34] , [35] . Thus, in regard to the cell lineage and signalling necessary for differentiation, the anterior PNS neurons and the dorsal PNS neurons in Ciona larvae are reminiscent of PNS neurons in vertebrate embryos, whereas the ventral PNS neurons are reminiscent of PNS neurons in cephalochordate and protostome embryos. Given that the innovation of neural crest cells and placodes is thought to be a key event in the course of evolution from primitive invertebrate chordates to vertebrates [32] , [36] , it is possible that the Ciona embryo might have both vertebrate-type and invertebrate-type PNS neurons. In the present study, we dissect a gene circuit involved in differentiation of ventral ESNs in the Ciona embryo, and compare it with a gene circuit involved in differentiation of dorsal ESNs for understanding evolution of PNSs in chordates. BMP signalling in the ventral ectodermal region Previous studies showed that the ventral ectodermal region of the tail is induced by a BMP ligand, Admp [16] , [25] . To determine when and where this signalling works, we used an antibody against phosphorylated Smad1/5/8 (pSmad1/5/8). To confirm that this antibody is immunoreactive against pSmad1/5/8 in ascidian embryos, we first stained early-tailbud embryos, in which BMP signalling is active in the ventral trunk region [37] . As shown in Fig. 1g , we detected strong pSmad1/5/8 staining in the ventral trunk region. In addition, when Bmp2/4 was overexpressed in the entire epidermis using the Dlx.b upstream region, pSmad1/5/8 staining was detected in the entire epidermis ( Supplementary Fig. 2a,c ). Conversely, when Noggin, which is an antagonist for BMP ligands, was overexpressed, pSmad1/5/8 staining was barely detectable ( Supplementary Fig. 2b,d ). Thus, this antibody successfully detected pSmad1/5/8 in ascidian embryos. 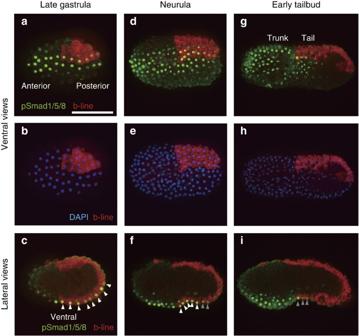Figure 1: BMP signalling is active in the ventral ectoderm from the late-gastrula to the tailbud stages. One of the posterior animal cells of eight-cell embryos were labelled with DiI (red) to show the anterior–posterior boundary and left–right boundary. (a,c,d,f,g,i) BMP signalling was detected with an antibody against phosphorylated Smad1/5/8 (green). (b,e,h) DAPI staining shows nuclei (blue) of the embryos shown ina,dandg. Ventral views are shown ina,b,d,e,gandh, and lateral views are shown inc,fandi. Photographs are Z-projected image stacks overlaid in pseudocolour. White and grey arrowheads inc,fandiindicate strong and weak signals, respectively. Scale bar, 100 μm (a). DAPI, 4,6-diamidino-2-phenylindole. Figure 1: BMP signalling is active in the ventral ectoderm from the late-gastrula to the tailbud stages. One of the posterior animal cells of eight-cell embryos were labelled with DiI (red) to show the anterior–posterior boundary and left–right boundary. ( a , c , d , f , g , i ) BMP signalling was detected with an antibody against phosphorylated Smad1/5/8 (green). ( b , e , h ) DAPI staining shows nuclei (blue) of the embryos shown in a , d and g . Ventral views are shown in a , b , d , e , g and h , and lateral views are shown in c , f and i . Photographs are Z-projected image stacks overlaid in pseudocolour. White and grey arrowheads in c , f and i indicate strong and weak signals, respectively. Scale bar, 100 μm ( a ). DAPI, 4,6-diamidino-2-phenylindole. Full size image As shown in Fig. 1a–c , we observed strong pSmad1/5/8 staining in two lines of cells of the ventral ectoderm from the anterior to the posterior end at the late-gastrula stage. We labelled one of two b4.2 blastomeres of the eight-cell embryo with DiI to identify the anterior–posterior border, because the tail ectoderm is derived from a pair of b4.2 cells. The tail region contained eight pSmad1/5/8-positive rows ( Fig. 1c ). At the neurula stage after the next cell division (10th division; most cells divide laterally), we detected pSmad1/5/8 in the anterior rows within the b4.2-line ectodermal cells and in the ventral ectodermal region of the trunk ( Fig. 1d–f ). The anterior five rows in the b4.2-line ectoderm contained a strong signal, and two or three additional rows contained a weaker signal. At the early-tailbud stage after the next cell division (11th division; most cells divide along the anterior–posterior axis), we detected a weak pSmad1/5/8 signal in only three anterior rows of the b4.2-line ectodermal cells ( Fig. 1g–i ). Indeed, pSmad1/5/8 staining at the late-gastrula stage was lost in embryos injected with a morpholino antisense oligonucleotide (MO) against Admp ( Fig. 2b,d ), while it was not affected in control embryos injected with a control MO against Escherichia coli lacZ ( Fig. 2a,c ). Bmp2/4 is activated by Admp signalling in the ventral trunk epidermis at the tailbud stage [37] , and begins to be expressed in the ventral epidermis at the late-gastrula stage [26] . We examined whether the expression of Bmp2/4 at the late-gastrula stage is also induced by Admp, and found that Bmp2/4 expression was lost in Admp morphants ( Fig. 2e,f ). Because Smad1/5/8 may be phosphorylated and activated by Bmp2/4 in addition to Admp, we collectively call signalling of Bmp2/4 and Admp as BMP signalling hereafter. 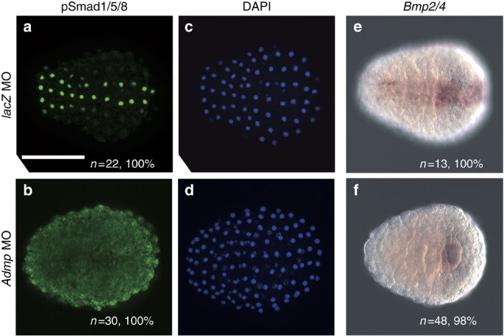Figure 2:Admpactivates Bmp signalling andBmp2/4expression in the ventral ectoderm at the late-gastrula stage. (a,b) BMP signalling was detected with an antibody against phosphorylated Smad1/5/8 (green) (a) in an embryo injected with a controlLacZMO, and (b) in an embryo injected with anAdmpMO. (c,d) DAPI staining shows nuclei (blue) of the embryos shown inaandb. (e,f) Expression ofBmp2/4at the late-gastrula stage is observed in the ventral ectoderm in an embryo injected with a controlLacZMO (e), while it is lost in an embryo injected with anAdmpMO (f). Scale bar, 100 μm (a). The number of embryos examined and the proportion of embryos that each panel represents are shown within the panels. DAPI, 4,6-diamidino-2-phenylindole. Figure 2: Admp activates Bmp signalling and Bmp2/4 expression in the ventral ectoderm at the late-gastrula stage. ( a , b ) BMP signalling was detected with an antibody against phosphorylated Smad1/5/8 (green) ( a ) in an embryo injected with a control LacZ MO, and ( b ) in an embryo injected with an Admp MO. ( c , d ) DAPI staining shows nuclei (blue) of the embryos shown in a and b . ( e , f ) Expression of Bmp2/4 at the late-gastrula stage is observed in the ventral ectoderm in an embryo injected with a control LacZ MO ( e ), while it is lost in an embryo injected with an Admp MO ( f ). Scale bar, 100 μm ( a ). The number of embryos examined and the proportion of embryos that each panel represents are shown within the panels. DAPI, 4,6-diamidino-2-phenylindole. Full size image Tbx2/3 is required for Msx expression in the ventral region Msx is important for differentiation of the dorsal ESNs [24] , [25] , and is also expressed in the ventral tail ectoderm [26] , suggesting that Msx is also important for differentiation of the ventral ESNs. To confirm this possibility, we injected a MO against Msx into fertilized eggs. In the resultant morphant embryos, Pou4 and Celf3.a ( Etr-1 ), which mark ESNs [26] , [38] (see Fig. 7c,e ), were not expressed ( Supplementary Fig. 3a,b ) in dorsal and ventral ESNs, except in a few ESNs near the tip of the tail. Because Msx is not expressed in the most posterior region, it is not surprising that ESNs near the tip of the tail of Msx morphants expressed Pou4 and Celf3.a . We also found that Pou4 and Celf3.a were ectopically expressed, when Msx was overexpressed in the entire epidermis using the Dlx.b upstream region ( Supplementary Fig. 3c,d ). Figure 7: Ascl.b and Tox regulate Delta.b , Pou4 and Celf3.a , which mark ESNs. Expression of ( a , b ) Delta.b , ( c , d ) Pou4 and ( e , f ) Celf3.a marks the ESNs (black arrowheads) ( a , c , e ) in control embryos injected with the control LacZ MO, but is completely lost ( b , d , f ) in double morphants of Ascl.b and Tox . Lateral views are shown. Note that three spots seen near the tip of the tail in f are cells of the nerve cord, but not ESNs. 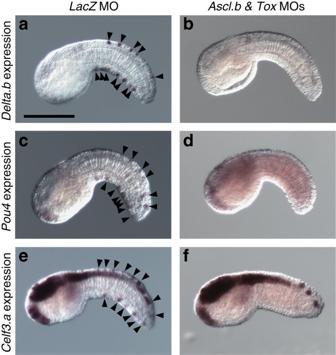Figure 7:Ascl.bandToxregulateDelta.b,Pou4andCelf3.a, which mark ESNs. Expression of (a,b)Delta.b, (c,d)Pou4and (e,f)Celf3.amarks the ESNs (black arrowheads) (a,c,e) in control embryos injected with the controlLacZMO, but is completely lost (b,d,f) in double morphants ofAscl.bandTox. Lateral views are shown. Note that three spots seen near the tip of the tail infare cells of the nerve cord, but not ESNs. Full size image A previous study showed that expression of Celf3.a in the ventral ESNs is under the control of BMP signalling [16] . In the present study, we found that expression of Msx in ventral tail ectoderm was similarly downstream of BMP signalling, because Msx expression in ventral tail ectoderm was upregulated in embryos overexpressed with Bmp2/4 using the Dlx.b enhancer, and downregulated in embryos overexpressed with Noggin ( Fig. 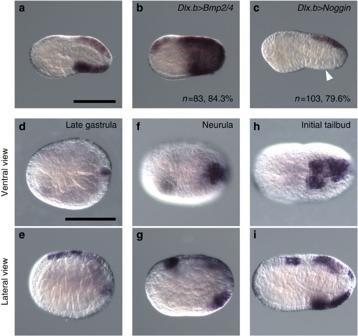3a–c ). Figure 3:Msxis under the control of Bmp signalling, and begins to be expressed in the ventral tail ectoderm at the neurula stage. (a–c)Msxexpression (a) in a control early-tailbud embryo, (b) in an embryo withBmp2/4overexpression under theDlx.benhancer and (c) in an embryo withNogginoverexpression under theDlx.benhancer. The white arrowhead indicates the region in whichMsxexpression is lost. The number of embryos examined and the proportion of embryos that each panel represents are shown within the panels. (d–i)Msxexpression (d,e) at the late-gastrula stage, (f,g) neurula stage and (h,i) initial-tailbud stage. (d,f,h) Ventral views and (e,g,i) lateral views are shown. Scale bar, 100 μm (a,d). Figure 3: Msx is under the control of Bmp signalling, and begins to be expressed in the ventral tail ectoderm at the neurula stage. ( a – c ) Msx expression ( a ) in a control early-tailbud embryo, ( b ) in an embryo with Bmp2/4 overexpression under the Dlx.b enhancer and ( c ) in an embryo with Noggin overexpression under the Dlx.b enhancer. The white arrowhead indicates the region in which Msx expression is lost. The number of embryos examined and the proportion of embryos that each panel represents are shown within the panels. ( d – i ) Msx expression ( d , e ) at the late-gastrula stage, ( f , g ) neurula stage and ( h , i ) initial-tailbud stage. ( d , f , h ) Ventral views and ( e , g , i ) lateral views are shown. Scale bar, 100 μm ( a , d ). Full size image We next investigated whether Msx began to be expressed at the same stage as Bmp2/4 , which is activated by Admp signalling, as described above. Although the expression pattern of Msx has been previously described [26] , [39] , we again examined Msx expression to determine the exact timing of its expression in ventral ectodermal cells ( Fig. 3d–i ). Msx was not expressed in the ventral ectoderm at the late-gastrula stage, and began to be expressed in the posterior half of the ventral tail ectoderm at the neurula stage. At the initial-tailbud stage, Msx was expressed in the entire ventral region of the tail ectoderm. Thus, because its expression initiates later than that of Bmp2/4 , Msx is not likely to be a direct target of Admp signalling. To identify candidate genes that are directly regulated by Admp signalling and regulate Msx expression, we used RNA sequencing (RNA-seq) to compare gene expression in late-gastrula embryos treated with recombinant BMP4 or a BMP inhibitor, dorsomorphin. Five transcription factor genes, including Msx , were greatly upregulated in embryos treated with BMP4 and downregulated in embryos treated with dorsomorphin ( Fig. 4a ). Nkxtun1 (formerly Nkx-A ) and NK2-3/5/6 (formerly NK4 ) are expressed specifically in ventral epidermis of the trunk at the tailbud stage, whereas Atoh8 (formerly Net ) is not specifically expressed in the ventral epidermis [26] . On the other hand, Tbx2/3 is expressed in the ventral ectoderm of the tail [26] , [40] , [41] . We therefore determined the exact timing of the initiation and termination of Tbx2/3 expression ( Fig. 4b–g ). At the late-gastrula stage, Tbx2/3 was expressed in the entire ventral ectoderm ( Fig. 4b,c ). At the neurula stage, expression of Tbx2/3 was diminished in the posterior half of the tail ectoderm, and became weaker in the rest of the ventral ectoderm ( Fig. 4d,e ). At the early-tailbud stage, expression of Tbx2/3 vanished completely in the ventral tail ectoderm ( Fig. 4f,g ). Thus, expression of Tbx2/3 preceded Msx expression. Tbx2/3 was indeed activated by Bmp signalling, as demonstrated by the observation that it was ectopically expressed in Bmp2/4 -overexpressing embryos ( Fig. 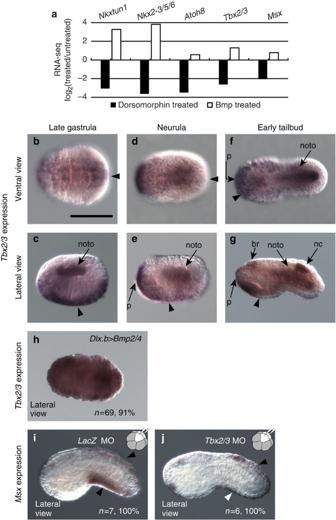4h ). Figure 4:Tbx2/3is expressed under Bmp signalling and regulatesMsxexpression in the ventral ectoderm. (a) RNA-seq experiments identified five transcription factor genes greatly upregulated and downregulated in embryos treated with Bmp4 and dorsomorphin, respectively (Pvalues adjusted for multiple testing <0.01, which were calculated by DEseq52; numbers of sequencing tags for untreated control embryos, Bmp4-treated embryos and dorsomorphin-treated embryos were 17,408,671, 10,657,653 and 16,157,915, respectively). (b–g)Tbx2/3expression (b,c) at the late-gastrula stage, (d,e) neurula stage and (f,g) early-tailbud stage. Expression in the ventral ectoderm is indicated by arrowheads. Note thatTbx2/3is also expressed in the notochord (noto), nerve cord (nc), brain (br) and palps (p). (h)Tbx2/3expression is expanded throughout the entire epidermal region of embryos withBmp2/4overexpression under the control of the upstream sequence ofDlx.b. (i,j) MOs against (i)LacZand (j)Tbx2/3were injected into the left and right posterior animal cells (b4.2) of eight-cell embryos. WhileMsxexpression was not affected (i) in embryos injected with theLacZMO and (j) in the dorsal region ofTbx2/3morphant embryos (black arrowheads), it was greatly reduced in the ventral region ofTbx2/3morphant embryos (white arrowhead). Scale bar, 100 μm (b). The number of embryos examined and the proportion of embryos that each panel represents are shown inh–j. All embryos are shown with anterior to the left. Figure 4: Tbx2/3 is expressed under Bmp signalling and regulates Msx expression in the ventral ectoderm. ( a ) RNA-seq experiments identified five transcription factor genes greatly upregulated and downregulated in embryos treated with Bmp4 and dorsomorphin, respectively ( P values adjusted for multiple testing <0.01, which were calculated by DEseq [52] ; numbers of sequencing tags for untreated control embryos, Bmp4-treated embryos and dorsomorphin-treated embryos were 17,408,671, 10,657,653 and 16,157,915, respectively). ( b – g ) Tbx2/3 expression ( b , c ) at the late-gastrula stage, ( d , e ) neurula stage and ( f , g ) early-tailbud stage. Expression in the ventral ectoderm is indicated by arrowheads. Note that Tbx2/3 is also expressed in the notochord (noto), nerve cord (nc), brain (br) and palps (p). ( h ) Tbx2/3 expression is expanded throughout the entire epidermal region of embryos with Bmp2/4 overexpression under the control of the upstream sequence of Dlx.b . ( i , j ) MOs against ( i ) LacZ and ( j ) Tbx2/3 were injected into the left and right posterior animal cells (b4.2) of eight-cell embryos. While Msx expression was not affected ( i ) in embryos injected with the LacZ MO and ( j ) in the dorsal region of Tbx2/3 morphant embryos (black arrowheads), it was greatly reduced in the ventral region of Tbx2/3 morphant embryos (white arrowhead). Scale bar, 100 μm ( b ). The number of embryos examined and the proportion of embryos that each panel represents are shown in h – j . All embryos are shown with anterior to the left. Full size image Next, we injected a Tbx2/3 MO into both of the left and right b4.2 blastomeres at the eight-cell stage to confirm that Tbx2/3 regulated Msx in the tail ectoderm cell-autonomously [26] (we did not injected the MO into fertilized eggs, because Tbx2/3 is also expressed in non-b-line cells). In these Tbx2/3 morphants, Msx expression was downregulated in the ventral tail ectoderm of tailbud embryos, but was unaffected in the dorsal tail ectoderm ( Fig. 4i,j ). For a further confirmation, the Tbx2/3 MO was injected into one of the posterior animal cells of eight-cell embryos (b4.2), Msx expression was lost in the ventral region on the injected side ( Supplementary Fig. 4a,b ). Thus, BMP signalling activates Tbx2/3 in the ventral tail ectoderm at the late-gastrula stage, and Tbx2/3 is required for activating Msx . Although Tbx2/3 is required for Msx expression in the ventral tail ectoderm, it might be insufficient for Msx expression. This is because Tbx2/3 messenger RNA (mRNA) injection into fertilized eggs failed to evoke ectopic expression of Msx ( Supplementary Fig. 5 ). BMP signalling itself or unidentified factors downstream of BMP signalling, together with Tbx2/3 , might work to activate Msx . Ascl.b and Tox are activated by Msx in the tail ectoderm Because Ascl.b (achaete-scute family bHLH transcription factor-b; formerly Ash2 ) and Tox ( TOX high-mobility group box family member; formerly CAGF9 ) are activated downstream of Msx in the dorsal ectoderm, where dorsal ESNs differentiate [25] , and because these two genes are also expressed in ventral tail ectoderm [26] , we investigated the possibility that Msx regulates the expression of these two genes in the ventral tail ectoderm. Expression of these two genes in the ventral tail ectoderm was not detectable at the late-gastrula or neurula stage, and began at the tailbud stage in normal embryos ( Fig. 5a–l ). These genes were strongly expressed in the ventral tail ectoderm, except for several cells near the trunk–tail border at the initial-tailbud stage. At the early-tailbud stage, both genes began to be expressed throughout the tail ventral ectoderm. 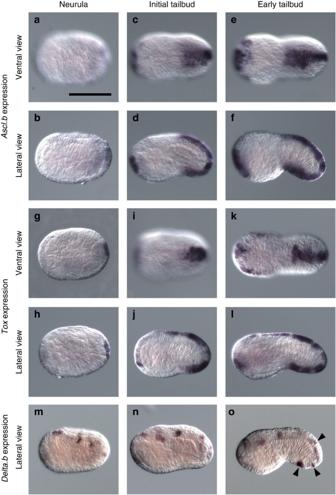Thus, expression of Ascl.b and Tox began later than Msx expression. Figure 5:Ascl.bandToxexpression begins at the initial-tailbud stage and precedesDelta.bexpression. (a–h) Expression of (a–f)Ascl.b, (g–l)Toxand (m–o)Delta.b. (a,b,g,h,m) at the neurula stage, and (c,d,i,j,n) initial-tailbud stage, and (e,f,k,l,o) early-tailbud stage. (a,c,e,g,i,k) Ventral views and (b,d,f,h,j,l–o) lateral views are shown. Prospective ESNs are indicated by black arrowheads ino. Scale bar, 100 μm (a). Figure 5: Ascl.b and Tox expression begins at the initial-tailbud stage and precedes Delta.b expression. ( a – h ) Expression of ( a – f ) Ascl.b , ( g – l ) Tox and ( m – o ) Delta.b . ( a , b , g , h , m ) at the neurula stage, and ( c , d , i , j , n ) initial-tailbud stage, and ( e , f , k , l , o ) early-tailbud stage. ( a , c , e , g , i , k ) Ventral views and ( b , d , f , h , j , l – o ) lateral views are shown. Prospective ESNs are indicated by black arrowheads in o . Scale bar, 100 μm ( a ). Full size image We first confirmed that injection of the control MO did not affect expression of Ascl.b and Tox ( Fig. 6a,b ). Next, we injected a MO against Tbx2/3 into both of the left and right b4.2 blastomeres. In the resultant morphant embryos, expression of Ascl.b and Tox in the tail ventral ectoderm was greatly reduced, whereas expression of the two genes in the dorsal ectoderm, in which Tbx2/3 was not expressed, was not affected ( Fig. 6c,d ). Likewise, the Tbx2/3 MO was injected into one of the posterior animal cells of eight-cell embryos (b4.2); expression of Ascl.b and Tox was lost in the ventral region on the injected side ( Supplementary Fig. 4c–f ). In Msx morphants, the expression of Ascl.b and Tox in the dorsal and ventral ectoderm, except for a few cells near the tip of the tail, was also lost ( Fig. 6e,f ). 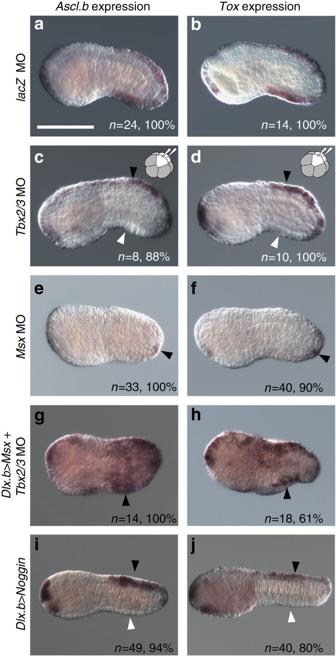Thus, the expression of Ascl.b and Tox in the dorsal ectoderm is under the control of Msx but not Tbx2/3 , while the expression in ventral ectoderm is under the control of Tbx2/3 and Msx . Figure 6:Ascl.bandToxare under the control ofTbx2/3,Msxand Bmp signalling. (a,b) Injection of the controlLacZMO into fertilized eggs did not affect the expression of (a)Ascl.bor (b)Tox. (c,d) When theTbx2/3MO was injected into the left and right posterior animal cells (b4.2) of eight-cell embryos, the expression of (c)Ascl.band (d)Toxwas greatly reduced in the ventral region (white arrowhead), but not in the dorsal region (black arrowhead). (e,f) The expression of (e)Ascl.band (f)Toxin both the ventral and dorsal regions was lost inMsxmorphants, except for a few cells in the posterior-most region (black arrowheads). (g,h) When theTbx2/3MO was injected into the left and right posterior animal cells (b4.2) of eight-cell embryos after electroporation of an overexpression construct forMsx, the expression of (g)Ascl.band (h)Toxwas observed in the ventral region (arrowheads) and the lateral epidermal region. With this construct,Msxwas overexpressed in the entire epidermis under the control of the upstream sequence ofDlx.b. Note that not all epidermal cells overexpressMsxbecause of mosaic incorporation of the electroporated plasmid. (i,j) The expression of (i)Ascl.band (j)Toxwas lost in the ventral region (white arrowheads), but not in the dorsal region (black arrowheads), of embryos with Noggin overexpression under the control of the upstream sequence ofDlx.b. The number of embryos examined and the proportion of embryos that each panel represents are shown. Scale bar, 100 μm (a). Figure 6: Ascl.b and Tox are under the control of Tbx2/3 , Msx and Bmp signalling. ( a , b ) Injection of the control LacZ MO into fertilized eggs did not affect the expression of ( a ) Ascl.b or ( b ) Tox . ( c , d ) When the Tbx2/3 MO was injected into the left and right posterior animal cells (b4.2) of eight-cell embryos, the expression of ( c ) Ascl.b and ( d ) Tox was greatly reduced in the ventral region (white arrowhead), but not in the dorsal region (black arrowhead). ( e , f ) The expression of ( e ) Ascl.b and ( f ) Tox in both the ventral and dorsal regions was lost in Msx morphants, except for a few cells in the posterior-most region (black arrowheads). ( g , h ) When the Tbx2/3 MO was injected into the left and right posterior animal cells (b4.2) of eight-cell embryos after electroporation of an overexpression construct for Msx , the expression of ( g ) Ascl.b and ( h ) Tox was observed in the ventral region (arrowheads) and the lateral epidermal region. With this construct, Msx was overexpressed in the entire epidermis under the control of the upstream sequence of Dlx.b . Note that not all epidermal cells overexpress Msx because of mosaic incorporation of the electroporated plasmid. ( i , j ) The expression of ( i ) Ascl.b and ( j ) Tox was lost in the ventral region (white arrowheads), but not in the dorsal region (black arrowheads), of embryos with Noggin overexpression under the control of the upstream sequence of Dlx.b . The number of embryos examined and the proportion of embryos that each panel represents are shown. Scale bar, 100 μm ( a ). Full size image We also found that the expression of Ascl.b and Tox was recovered in the tail ventral ectoderm and observed ectopically in the head and tail ectoderm, when the Msx overexpression construct was introduced into fertilized eggs by electroporation and then the Tbx2/3 MO was injected into both of the left and right b4.2 blastomeres at the eight-cell stage ( Fig. 6g,h ). Therefore, Msx can activate Ascl.b and Tox in the absence of Tbx2/3 , and Tbx2/3 controls Ascl.b and Tox through activation of Msx. Finally, we examined the expression of Ascl.b and Tox in embryos with Noggin overexpression using the Dlx.b enhancer. In these embryos, the expression in the ventral tail ectoderm was specifically lost ( Fig. 6i,j ). This observation confirmed that BMP signalling is required for genes activated in the ventral tail ectoderm. Tox and Ascl.b are required for differentiation of ESNs Delta.b is expressed in dorsal and ventral ESNs, and Delta.b signalling represses Pou4 and Celf3.a ( Etr-1 ) in the surrounding epidermal cells [16] , [24] , [42] . Delta.b expression in the ventral tail ectoderm begins in scattered cells of the posterior region and subsequently expands into the anterior tail region [16] . Through Delta/Notch–mediated lateral inhibition, the number of neurons are thought to be controlled [16] . We first investigated whether expression of Ascl.b and Tox preceded Delta.b expression in dorsal and ventral ESNs. Delta.b was not expressed in prospective ESNs at the neurula and initial-tailbud stages ( Fig. 5m,n ), and began to be expressed in prospective ESNs at the early-tailbud stage in the posterior region ( Fig. 5o ). At the middle-tailbud stage, prospective ESNs in the anterior tail region began to express Delta.b [16] (see also Fig. 7a ). Thus, initiation of Delta.b expression in prospective ESNs occurred one step later than initiation of Ascl.b and Tox expression. When we injected MOs against either of Ascl.b or Tox , expression of Delta.b , Pou4 and Celf3.a was lost or reduced in most embryos ( Table 1 ; Supplementary Fig. 6 ). In double morphants of Ascl.b and Tox , the expression of these three genes was almost completely lost ( Table 1 ; Fig. 7a–f ). Thus, Ascl.b and Tox are both required for differentiation of ESNs in the ventral and dorsal ectoderm. Table 1 Effects of knockdown of Ascl.b and Tox . Full size table A previous study reported that there are two morphologically distinct populations among the ESNs of the ventral tail ectoderm, because posterior ESNs have longer axons than anterior ESNs [43] . Our analysis showed that ESNs in the anterior and posterior halves of the ventral tail ectoderm use the same gene circuit beginning with BMP signalling, although timing of the initiation of Msx expression differs between the anterior and posterior populations. We showed that Tbx2/3 is required for Msx expression in the ventral ectoderm. Although Tbx2/3 and its orthologues, Tbx2 and Tbx3, often act as a repressor, Tbx2 and Tbx3 are also known to act as activators [44] , [45] . Therefore, it is not surprising that Tbx2/3 directly activates Msx in the ventral ectoderm, although it is also possible that Tbx2/3 acts as a repressor and indirectly activates Msx . We also showed that ventral and dorsal tail ESNs are specified by a common genetic pathway comprising Msx , Tox / Ascl.b and Delta.b / Celf3.a / Pou4 , whereas the upstream mechanism of Msx regulation differs between these two lineages ( Fig. 8 ). In the dorsal lineage, Otx and Nodal are required for Msx expression [24] , [25] , and these two genes are activated by a combination of the activating influence of FGF signalling and the repressive influence of Ephrin, Admp and Gdf1/3-r signalling at the 32-cell stage [17] , [18] , [19] , [20] , [21] , [22] . In the ventral lineage, BMP signalling induces Tbx2/3 at the late-gastrula stage, and this Tbx2/3 expression is required for Msx expression. Hence, the evidence that co-option of the gene circuit downstream of Msx created a novel lineage of ESNs is persuasive. If so, which of the lineages represents the original one? We favour the hypothesis that the ventral lineage is the original one, for two reasons. First, the ventral lineage is induced by BMP signalling, and PNS neurons in amphioxus and protostomes are also induced by BMP signalling [33] , [34] , [35] . Second, although cells giving rise to the dorsal ESNs in the ascidian embryos are embedded in the epidermis and not migratory, the dorsal lineage is derived from cells located at the border of the epidermal lineage and neural plate, reminiscent of the situation in vertebrate PNSs. 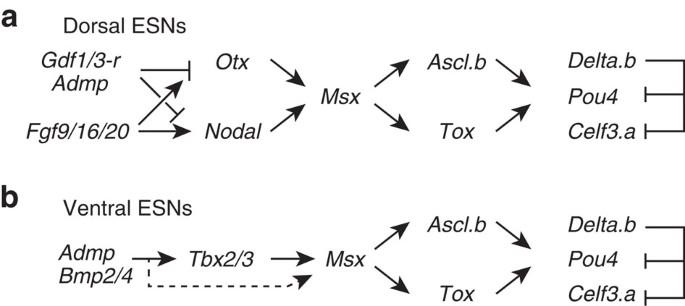Figure 8: Summary of the regulatory gene circuits involved in differentiation of the dorsal and ventral ESNs. (a) Dorsal ESNs and (b) ventral ESNs share a gene circuit downstream ofMsx, whereas the regulatory mechanisms upstream ofMsxdiffer between these two lineages. These circuits are based on the results of the present and previous studies16,24,25,43. BecauseTbx2/3alone failed to activateMsx, BMP signalling itself or unidentified factors downstream of BMP signalling, together withTbx2/3, might work to activateMsx(a dotted arrow). Figure 8: Summary of the regulatory gene circuits involved in differentiation of the dorsal and ventral ESNs. ( a ) Dorsal ESNs and ( b ) ventral ESNs share a gene circuit downstream of Msx , whereas the regulatory mechanisms upstream of Msx differ between these two lineages. These circuits are based on the results of the present and previous studies [16] , [24] , [25] , [43] . Because Tbx2/3 alone failed to activate Msx , BMP signalling itself or unidentified factors downstream of BMP signalling, together with Tbx2/3 , might work to activate Msx (a dotted arrow). Full size image In anamniote embryos, Rohon-Beard mechanosensory neurons are also formed from the neural plate border [5] . An anatomical study suggested that Retzius bipolar cells of amphioxus are homologous to Rohon-Beard sensory neurons [46] . It is possible that the ascidian dorsal ESNs are homologous to Rohon-Beard neurons, and this possibility is not necessarily mutually exclusive with the above possibility that the ascidian dorsal ESNs are homologous to vertebrate PNS neurons derived from neural crest cells. Indeed, the gene networks that specify Rohon-Beard neurons and the neural crest are overlapped considerably [47] . None of these scenarios is inconsistent with our hypothesis that a novel lineage of ESNs were born by co-option of the gene circuit downstream of Msx . In vertebrate embryos, BMP signalling negatively regulates neural fate during the initial process of neural induction, but later an intermediate level of BMP signalling is required for neural crest formation [48] , [49] . Msx is indeed a direct target of BMP signalling at the neural plate border [50] . However, because Msx may not be a direct target of BMP signalling in the ventral ectoderm of the ascidian embryo, the gene circuit comprising BMP signalling, Tbx2/3 and Msx in the ascidian embryo is not likely directly relevant with the gene circuit that activates Msx in vertebrate embryos. Taken together, the available data suggest that a common ancestor of Ciona and vertebrates acquired the secondary PNS lineage around the neural plate border by co-option of a gene circuit activated by Msx . Thus, the ventral ESNs of the ascidian larva may not be directly homologous to vertebrate PNSs, and the original lineage might have been lost in the vertebrates. In situ hybridization and immunostaining C. intestinalis adults were obtained from the National Bio-Resource Project for Ciona . Complementary DNA clones were obtained from our clone collection used for obtaining expressed sequence tags (ESTs) [51] . For whole-mount in situ hybridization, digoxigenin-RNA probes were synthesized by in vitro transcription with T7 RNA polymerase. Embryos were fixed in 4% paraformaldehyde in 0.1 M MOPS-NaOH (pH 7.5) and 0.5 M NaCl at 4 °C overnight and then stored in 80% ethanol. After a wash with PBS containing 0.1% tween 20 (PBST), embryos were treated with 2 μg ml −1 Protenase K for 30 min at 37 °C, washed again with PBST and fixed with 4% paraformaldehyde for 1 h at room temperature. Embryos were then incubated in 6 × saline sodium citrate buffer, 50% formamide, 5 × Denhardt’s solution, 100 μg ml −1 yeast tRNA and 0.1% tween 20 for 1 h at 50 °C. After this prehybridization step, specific RNA probes were added and incubated for 16 h at 50 °C. Embryos were treated with RNase A, and incubated in 0.5 × saline sodium citrate buffer, 50% formamide and 0.1% tween 20 for 15 min at 50 °C twice. Embryos were further incubated in 0.5% blocking reagent (Roche) in PBST for 30 min, and then in 1:2,000 alkaline-phosphatase-conjugated anti-digoxigenin antibody (Roche). After a PBST wash, embryos were further washed with 0.1 M NaCl, 50 mM MgCl 2 and 0.1 M Tris-HCl (pH 9.5), and then p-nitroblue tetrazolium chloride (NBT) and 5-bromo-4-chloro-3-indolyl phosphate (BCIP) were used for detection. To detect activation of the Bmp signalling pathway, embryos were fixed with 3.7% formaldehyde in PBS, treated with 3% H 2 O 2 for 30 min and then incubated with a rabbit polyclonal antibody against a synthetic phosphopeptide derived from human Smad1 (Abcam, ab97689; 1:1,000; Ciona Smad1/5/8 has the same amino-acid sequence in its C-terminal end) in Can-Get-Signal-Immunostain Solution B (Toyobo). The signal was visualized with a TSA kit (Invitrogen) using horseradish peroxidase-conjugated goat anti-rabbit immunoglobulin-G and Alexa Fluor 488 tyramide. For RNA-seq experiments, embryos were treated with human BMP4 (100 ng ml −1 ; HumanZyme) and dorsomorphin (100 μM; Wako) continuously after fertilization, and collected at the late-gastrula stage. RNA-seq experiments were performed using the Illumina TruSeq RNA Sample Preparation kit and the Illumina Hiseq2500 sequencer. We did not take duplicates, mainly because we used this experiment for screening, and the obtained result was confirmed with other methods. Sequence data are deposited in the SRA database under the accession numbers, DRR033088–DRR033090. DEseq was used to identify differentially expressed genes [52] . Identifiers for genes examined in the present study are as follows: CG.KH2012.C2.421 for Admp , CG.KH2012.C4.125 for Bmp2/4 , CG.KH2012.C12.562 for Noggin , CG.KH2012.L96.87 for Tbx2/3 , CG.KH2012.C2.957 for Msx , CG.KH2012.C12.577 for Nkxtun.a ( Nkx-A ), CG.KH2012.C8.482 for Nkx2-3/5/6 ( NK4 ), CG.KH2012.C9.872 for Atho8 ( Net ), CG.KH2012.L9.13 for Ascl.b , CG.KH2012.C3.330 for Tox , CG.KH2012.L50.6 for Delta.b , CG.KH2012.C2.42 for Pou4 and CG.KH2012.C6.128 for Celf3.a . Gene knockdown and overexpression The MOs (Gene Tools, LLC) against LacZ , Admp , Tbx2/3 and Msx , which block translation, were used previously [25] , [53] ; LacZ , 5′-TACGCTTCTTCTTTGGAGCAGTCAT-3′; Admp , 5′-TATCGTGTAGTTTGCTTTCTATATA-3′; Tbx2/3 , 5′-GAGGTCCACACCAACACTTTAACAT-3′; Msx , 5′-ATTCGTTTACTGTCATTTTTAATTT-3′. We designed an additional MO against Tbx2/3 (5′-GGTCTTCGCTATCGGTCAAACACAT-3′). Because two Tbx2/3 MOs yielded the same phenotype (downregulation of Msx ; Supplementary Fig. 7a ), only results obtained with the first MO are shown, unless otherwise noted. We also designed one MO that blocks translation (5′-CATCGTCCATCATAAGTTGTAGCAT-3′) and one MO that blocks splicing of Tox (5′-TGTCCCTGGAGAATCGGCGAATCAA-3′). Because both MOs yielded the same phenotype (downregulation of Pou4 and Celf3.a ; Supplementary Fig. 7b,c ), only results obtained with the first MO are shown, unless otherwise noted. Although we designed two MOs that block translation of Ascl.b (5′-GCGGTTCGTCACTTCCGGTCGCCAT-3′ and 5′-TCACTTCCGGTCGCCATTTTTGTTC-3′), the second one yielded a nonspecific phenotype; embryos injected with the second MO started to be disorganized at the eight-cell stage. However, we believe that the data obtained with the first MO are specific, because overexpression of Ascl.b gave opposite phenotypes (ectopic expression of Pou4 and Celf3.a ; Supplementary Fig. 7d,e ), because Gfp gene, in which the first codon (ATG) was replaced with a nucleotide sequence including an Ascl.b MO target site (5′-ATGGCGACCGGAAGTGACGAACCGCGG-3′), was not expressed by coinjection with the Ascl.b MO ( Supplementary Fig. 7f,g ), and because phenotypes of double morphants of Ascl.b and Tox were stronger than those of single morphants of either of Ascl.b or Tox . MOs were introduced by microinjection under a microscope. All experiments were repeated at least twice with different batches of embryos. The DNA constructs used for overexpression of Msx , Bmp2/4 and Noggin under the Dlx.b upstream sequence (Ciinte.REG.KH.C7.630497–632996| Dlx.b ) were used previously [37] . These DNA constructs were introduced by electroporation. For mRNA injection experiments, in vitro synthesized capped mRNA for Tbx2/3 was prepared using an mMESSAGE mMACHINE T3 Transcription kit (Life Technologies). All experiments were repeated at least twice with different batches of embryos. Accession codes: RNA-seq data generated in this study have been deposited in the SRA database under the accession codes DRR033088 – DRR033090 . How to cite this article: Waki, K. et al. Genetic pathways for differentiation of the peripheral nervous system in ascidians. Nat. Commun. 6:8719 doi: 10.1038/ncomms9719 (2015).